Self-healing of quantum entanglement after an obstruction Quantum entanglement between photon pairs is fragile and can easily be masked by losses in transmission path and noise in the detection system. When observing the quantum entanglement between the spatial states of photon pairs produced by parametric down-conversion, the presence of an obstruction introduces losses that can mask the correlations associated with the entanglement. Here we show that we can overcome these losses by measuring in the Bessel basis, thus once again revealing the entanglement after propagation beyond the obstruction. We confirm that, for the entanglement of orbital angular momentum, measurement in the Bessel basis is more robust to these losses than measuring in the usually employed Laguerre–Gaussian basis. Our results show that appropriate choice of measurement basis can overcome some limitations of the transmission path, perhaps offering advantages in free-space quantum communication or quantum processing systems. Quantum entanglement in the orbital angular momentum (OAM) modes of photons has been topical of late, promising to offer access to high-dimensional Hilbert spaces [1] . It was shown that beams with an azimuthal phase dependence exp( iℓφ ) carry an OAM of ℓ ħ per photon, where the azimuthal index ℓ can assume any integer value [2] . Laguerre–Gaussian (LG) modes are examples of such beams and are commonly used to exploit the OAM property of light [3] , [4] . As such, the LG modes were first used to demonstrate OAM entanglement [5] . However, a variety of bases may also be used to demonstrate OAM entanglement, including Ince–Gaussian [6] , Bessel–Gaussian (BG) [7] , [8] as well as mutually unbiased bases derived from these sets [9] , [10] . The OAM modal basis defines an infinite-dimensional Hilbert space, allowing access to high-dimensional entanglement [11] . An increase in dimension leads to improved security in quantum key distribution as well as increased information capacity in quantum communication protocols [12] , [13] . Unfortunately, while photons are weakly interacting, their entanglement is nevertheless fragile to the environment [14] . There have been a number of efforts in mitigating the decoherence in quantum computers and information processes based on ion traps, nuclear magnetic resonance and hyper-entanglement [15] , [16] , [17] . There have also been theoretical suggestions to recover lost entanglement [18] ; however, it is yet to be demonstrated experimentally. In the context of OAM modes, the decay of entanglement has been both predicted [19] and measured [20] for atmospheric turbulence as an environment, with some success in diminishing these effects [21] , [22] , [23] . Here we investigate the ability of OAM modes to recover the measured degree of entanglement of the quantum state after encountering an obstruction. It is well known that BG beams have the ability to self-heal after encountering an obstruction [24] , [25] . An obstruction placed in the path of one of the down-converted photons introduces an optical loss such that the OAM entanglement, as witnessed by the Clauser Horne Shimony Holt (CHSH) inequality, is obscured. We then show that by measuring in the BG basis the classical self-healing of the Bessel profile gives a higher signal and the OAM entanglement is once again revealed. We demonstrate a dependence of the calculated concurrence of the quantum state on the location of the obstruction within the propagation path, and find that this is in agreement with the classical self-healing distance of BG beams. We thus find that even when applied to single photons this self-healing property of the Bessel beam allows us to overcome the losses associated with the obstruction such that the spatial correlations can be measured with sufficient fidelity to reveal the quantum entanglement of the photon pairs. Bessel beams Bessel beams represent a class of nominally propagation-invariant solutions to the Helmholtz equation [26] and have been extensively investigated to date [27] . A laboratory approximation to these fields, BG beams, has similar properties over finite distances [28] , including their ability to reconstruct both in amplitude and phase after encountering an obstruction [24] , [25] . Although this property has been studied using classical light and single photons [29] , it may also be applicable in quantum processes. Higher-order Bessel and BG beams have helical wavefronts and carry OAM [30] . Entanglement of the OAM modes in the BG basis has been shown to offer a wider spiral spectrum as compared with the LG basis [7] . A BG beam is a superposition of plane waves with wave vectors that lie on a cone [28] . The electric field of a scalar BG mode of order ℓ is given by where ℓ is the azimuthal (mode) index (a signed integer); J ℓ (·) is the Bessel function of the first kind; k r and k z are the radial and longitudinal wave vectors, respectively. The initial radius of the Gaussian profile is w 0 and the Rayleigh range is z R = π / λ , where λ is the wavelength of the BG mode. A BG beam has a finite propagation distance, z max , over which it is said to be nominally non-diffracting [27] , shown as the shaded diamond-like region in Fig. 1 . In this region the incoming plane waves are refracted through an axicon (conical lens) and interfere to form the BG beam. The resulting wave vectors lie on a cone of angle θ =arcsin( k r / k ). Using simple geometric arguments, the maximum propagation distance is defined as z max =2 πw 0 / λk r , where sin( θ )≈ θ for small θ . If an obstruction of radius R is placed in the BG field, a shadow region is formed (see Fig. 1 ). However, those plane waves that bypass the obstruction will again interfere to form a BG beam [24] , [25] . 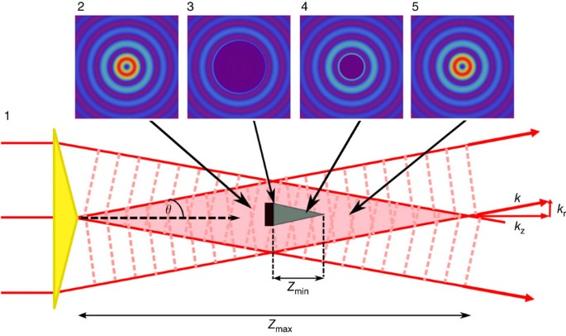Figure 1: Self-healing property of BG beams. The BG beam is generated using a computer-generated hologram of an axicon (yellow triangle) and exists in a finite region,zmax(pink diamond). An obstacle placed in the centre of the BG region (black rectangle) obstructs the beam for a minimum distance,zmin(grey triangle), after which the BG field reforms. The insets display the expected image of the beam at four different planes. The distance after which the field will recover is given by Figure 1: Self-healing property of BG beams. The BG beam is generated using a computer-generated hologram of an axicon (yellow triangle) and exists in a finite region, z max (pink diamond). An obstacle placed in the centre of the BG region (black rectangle) obstructs the beam for a minimum distance, z min (grey triangle), after which the BG field reforms. The insets display the expected image of the beam at four different planes. Full size image and is determined from purely geometric arguments [31] . The insets in Fig. 1 show the effect of an obstruction on the expected BG field at different planes. We generate BG modes by encoding a phase-only hologram onto a spatial light modulator (SLM) [32] , [33] . The transmission function of this hologram is written as where sign{·} denotes the sign function. In the following experimental results, we generated a BG mode with k r =30 rad mm −1 . Our experimental setup, shown in Fig. 2 , consisted of a type-I crystal used to produce collinear, degenerate entangled pairs of photons via spontaneous parametric down-conversion (SPDC). A glass plate with a circular obstruction with a 200-μm radius was placed after the crystal in the path of the down-converted light and mounted on a z -axis translation stage. The plane of the crystal was imaged with a × 2 magnification onto two separate SLMs, where the state into which the photon was projected is defined. Each SLM plane was then imaged with a × 250 demagnification to the input of a single-mode fibre (SMF), which only allows the propagation of the fundamental mode. The SMFs were attached to avalanche photodiodes (APDs), which were in turn connected to a coincidence counter. 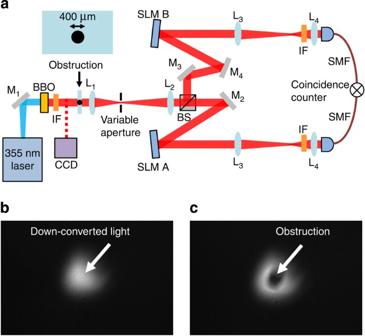Figure 2: Experimental setup. The setup shown was used to measure the effect of an obstruction in the path of the down-converted light. (a) An ultraviolet laser source pumped a type-I BBO crystal to produce pairs of entangled photons via SPDC. The crystal plane was imaged onto two separate SLMs using lenses L1(f1=200 mm) and L2(f2=400 mm). Each SLM plane was again imaged to the input of an SMF using lenses L3(f3=500 mm) and L4(f4=2 mm). (b) The down-converted beam at the plane of the crystal. (c) A circular obstruction (radius=200 μm) was placed between the crystal and lens L1, in the path of the down-converted light. Figure 2: Experimental setup. The setup shown was used to measure the effect of an obstruction in the path of the down-converted light. ( a ) An ultraviolet laser source pumped a type-I BBO crystal to produce pairs of entangled photons via SPDC. The crystal plane was imaged onto two separate SLMs using lenses L 1 ( f 1 =200 mm) and L 2 ( f 2 =400 mm). Each SLM plane was again imaged to the input of an SMF using lenses L 3 ( f 3 =500 mm) and L 4 ( f 4 =2 mm). ( b ) The down-converted beam at the plane of the crystal. ( c ) A circular obstruction (radius=200 μm) was placed between the crystal and lens L 1 , in the path of the down-converted light. Full size image Setup The experimental setup in Fig. 2 was first aligned in back-projection mode, where a classical laser source was connected to one of the SMFs to allow light to propagate through the system in reverse. Klyshko’s advanced-wave representation considered the field detected in arm A as propagating in reverse back to the crystal plane, where it reflects off the crystal to propagate forward through the system to detector B [34] . This method has been shown to be useful in examining the conditional probability distribution of the coincidence count rate [8] . We implemented this concept experimentally by disconnecting fibre A from one of the APDs and reconnecting it to a continuous light source at λ =710 nm. The classical light was directed onto SLM A and imaged to the crystal plane via lenses L 1 and L 2 . Images of the obstruction were recorded by placing a mirror between the crystal and obstruction and a CCD camera at the plane of the crystal. Classical images of the self-healing property are shown in Fig. 3 for both the BG ( Fig. 3a–d ) and LG ( Fig. 3e–h ) modes, where the unobstructed BG and LG modes are shown in (a) and (e), respectively. We calculated the maximum propagation distance of the BG field as z max =169.6 mm. The obstruction was first placed at the plane of the crystal, which is clearly shown in both (b) and (f). It was then moved 20 mm away from the crystal plane, shown in (c) and (g). The final images, (d) and (h), were taken 50 mm away from the crystal. It is clear that the BG mode has reformed at 50 mm, while the LG mode has not resumed its original structure. In a typical self-healing experiment [25] , the obstruction is placed at a fixed position in the path of the beam and the CCD camera is moved such that the subsequent planes behind the obstruction can be imaged. However, an identical effect is seen if the CCD camera remains fixed, imaging one particular plane, and the obstruction is moved away from that plane. This is illustrated in Fig. 4 , where we consider back-projected light directed from the SLM to the crystal. The obstruction is moved away from the crystal towards lens L 1 . As the obstruction moves, the shadow region falling on the crystal becomes less significant until finally it no longer falls on the crystal and the recovered mode is observed as shown in Fig. 3d . 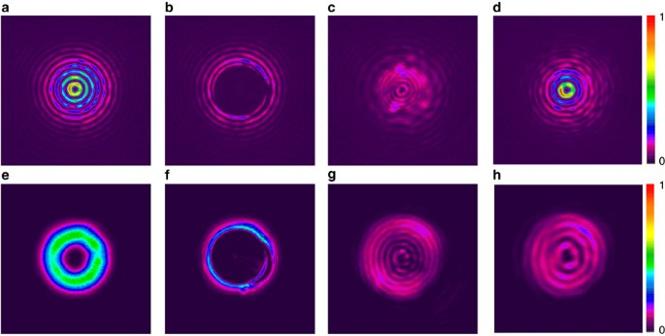Figure 3: CCD images of the crystal plane for different on-axis obstruction positions. Images for a BG mode (a–d) and an LG mode (e–h) with the azimuthal indexℓ=2. The unobstructed modes are shown in (a) and (e). The obstruction was first placed at the plane of the crystal, which is clearly shown in both (b) and (f). It was then moved 20 mm away from the crystal plane, shown in (c) and (g). The final images, (d) and (h), were taken 50 mm away from the crystal. It is clear the BG mode has reformed at 50 mm, while the LG mode has not resumed its original structure. Figure 3: CCD images of the crystal plane for different on-axis obstruction positions. Images for a BG mode ( a – d ) and an LG mode ( e – h ) with the azimuthal index ℓ =2. The unobstructed modes are shown in ( a ) and ( e ). The obstruction was first placed at the plane of the crystal, which is clearly shown in both ( b ) and ( f ). It was then moved 20 mm away from the crystal plane, shown in ( c ) and ( g ). The final images, ( d ) and ( h ), were taken 50 mm away from the crystal. It is clear the BG mode has reformed at 50 mm, while the LG mode has not resumed its original structure. 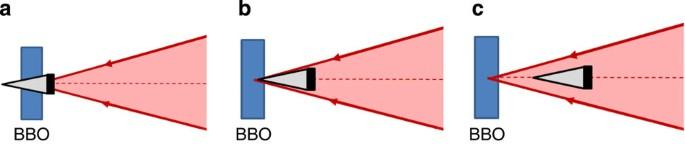Figure 4: Movement of the obstruction within the Bessel region. Consider the back-projected beam reflecting off the SLM onto the BBO crystal. The Bessel hologram on the SLM creates a beam with a particular cone angle. (a) The obstruction is at the closest position to the crystal, resulting in a clear shadow region falling on the crystal. (b) The obstruction is moved away from the crystal, reducing the shadow region. (c) The obstruction is moved further away such that the shadow region no longer falls on the crystal and a recovered BG image is seen (Fig. 3d). Full size image Figure 4: Movement of the obstruction within the Bessel region. Consider the back-projected beam reflecting off the SLM onto the BBO crystal. The Bessel hologram on the SLM creates a beam with a particular cone angle. ( a ) The obstruction is at the closest position to the crystal, resulting in a clear shadow region falling on the crystal. ( b ) The obstruction is moved away from the crystal, reducing the shadow region. ( c ) The obstruction is moved further away such that the shadow region no longer falls on the crystal and a recovered BG image is seen ( Fig. 3d ). Full size image From equation (2), we calculated a minimum self-healing distance of ~29 mm for R =200 μm and k r =30 rad mm −1 . After a distance, the obstructed BG mode demonstrated a restored structure, while the LG mode showed no self-healing. The BG field reconstructed after z min as expected. The setup was then returned to the down-conversion mode (both SMFs were connected to their respective detectors) to investigate the effects of the obstruction on two-photon quantum correlations. As OAM is conserved in SPDC [5] , we chose to first project the signal and idler photons into the | ℓ =±2› basis elements, respectively. The coincidence count rate of this BG state, unobstructed, was measured to be ~140 s −1 . The obstruction was initially inserted 5 mm after the β -barium borate (BBO) crystal, the closest it could be placed owing to the size of the crystal housing, and moved in subsequent intervals of 5 mm away from the crystal. Slight adjustments were made to the position of the obstruction until a minimum count rate was measured, causing the coincidence levels to be reduced to background levels. At each position coincidences were recorded; a comparison of the coincidence count rates for the BG and LG modes is shown in Fig. 5 . The count rate for the BG mode increased significantly after a distance of 25 mm, which is consistent with our calculation of z min =29 mm. Conversely, the count rates for the LG mode showed no measurable change with distance, illustrating the unique self-healing property of BG modes. The coincidence count rate of the BG mode was not restored to the original, unobstructed rate, as there is a loss due to the obstacle. This is also consistent with the classical scenario where the self-healed BG beam has proportionally less energy after the obstacle than before. 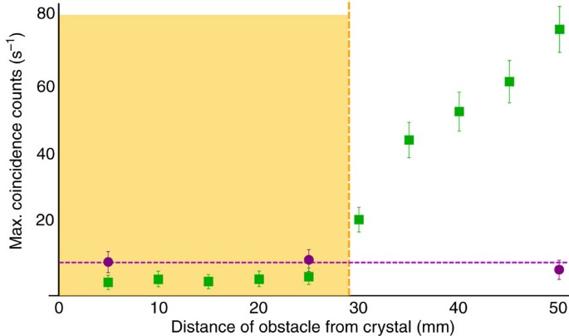Figure 5: Effect of an obstacle on the coincidence count rate. Measured coincidence count rates as a function of the position of the obstruction after the BBO crystal for a BG (green squares) and LG (purple circles) mode for |ℓ=±2› subspace. The BG mode withkr=30 rad mm−1is expected to reconstruct after an obstruction with radius,R=200 μm, after a distance of 29 mm (yellow dashed line). The coincidence count rate remains consistently low when measured in the LG basis (purple dashed line). The count rates were averaged over a set of 10 measurements, each taken over an integration period of 5 s. Errors were estimated assuming Poisson statistics for the photon counts given as an s.d. Figure 5: Effect of an obstacle on the coincidence count rate. Measured coincidence count rates as a function of the position of the obstruction after the BBO crystal for a BG (green squares) and LG (purple circles) mode for | ℓ =±2› subspace. The BG mode with k r =30 rad mm −1 is expected to reconstruct after an obstruction with radius, R =200 μm, after a distance of 29 mm (yellow dashed line). The coincidence count rate remains consistently low when measured in the LG basis (purple dashed line). The count rates were averaged over a set of 10 measurements, each taken over an integration period of 5 s. Errors were estimated assuming Poisson statistics for the photon counts given as an s.d. Full size image Measuring the degree of entanglement The recovery of the BG coincidence count rate does not in itself give an indication of the effects the obstruction has on the degree of entanglement of the state. To investigate the measured degree of entanglement, we first performed a Bell-type inequality experiment on the reformed state with the obstruction located 45 mm from the crystal to test for quantum correlations. The superposition of OAM states, also known as sector states, for | ℓ =±2› subspace were rotated on each SLM [35] and the corresponding coincidence count rates were recorded, shown in Fig. 6a . 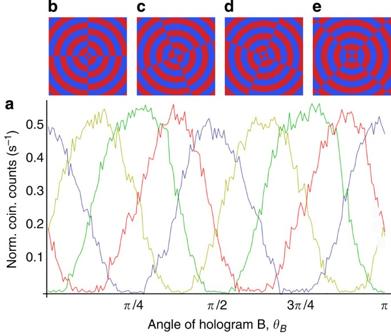Figure 6: CHSH-Bell measurements. (a) Normalized coincidence count rate as a function of the orientation of the hologram on SLM B. The hologram on SLM A was oriented at four different angles: 0 rad (blue curve),π/8 rad (yellow curve),π/4 rad (green curve) and 3π/8 rad (red curve). The measured count rates were normalized by the denominator in equation (5). The typical sinusoidal Bell curve was measured with the obstruction placed in the propagation path at 45 mm from the crystal. Examples of the binary Bessel holograms (|ℓ=±2›) used to perform a CHSH-inequality experiment are shown in the insets (b–e). Figure 6: CHSH-Bell measurements. ( a ) Normalized coincidence count rate as a function of the orientation of the hologram on SLM B. The hologram on SLM A was oriented at four different angles: 0 rad (blue curve), π /8 rad (yellow curve), π /4 rad (green curve) and 3 π /8 rad (red curve). The measured count rates were normalized by the denominator in equation (5). The typical sinusoidal Bell curve was measured with the obstruction placed in the propagation path at 45 mm from the crystal. Examples of the binary Bessel holograms (| ℓ =±2›) used to perform a CHSH-inequality experiment are shown in the insets ( b – e ). Full size image From the count rates we calculated the CHSH-Bell parameter to be S =2.78±0.04, which is a clear violation of the CHSH-Bell inequality [36] . This value of S can be compared with the unobstructed value of S =2.79±0.03. The low coincidence count rate recorded when the obstruction was 5 mm from the crystal resulted in a low-contrast Bell curve, from which the S parameter could not be calculated. This prompted us to perform a full-state tomography experiment [37] to determine the degree of entanglement of the state. 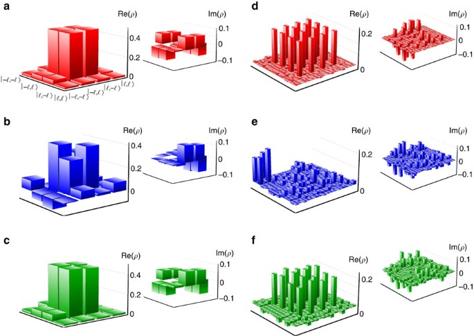Figure 7: Reconstructed density matrices from full-state tomography measurements. The density matrices are shown for dimensionsd=2 (a–c) andd=4 (d–f). Real and imaginary parts of the reconstructed density matrices for (a) and (d) no obstruction, (b) and (e) obstruction placed 5 mm from the crystal, and (c) and (f) obstruction placed 45 mm from the crystal. It is clear that the density matrix recovers to the original unobstructed form for a two-dimensional state as well as higher-dimensional states. The density matrices were calculated by measuring an over-complete set of modes and applying a maximum-likelihood estimation using a least-squares fit to the measurements. This optimization technique ensures a density matrix with non-negative eigenvalues and a trace of unity. Figure 7 shows the real and imaginary parts of the reconstructed density matrices for dimensions d =2 for | ℓ =±2› and d =4 for | ℓ ={−2, −1, 1, 2}›. The unobstructed density matrices for d =2 and d =4 are shown in Fig. 7a,d , respectively. When the obstruction is placed near the crystal, the density matrices in both cases change significantly such that the inner dominant probabilities are reduced and the outer terms become non-zero, Fig. 7b,e . However, once the obstruction is moved beyond the z min distance, both density matrices return to their original form ( Fig. 7c,f ). Figure 7: Reconstructed density matrices from full-state tomography measurements. The density matrices are shown for dimensions d =2 ( a – c ) and d =4 ( d – f ). Real and imaginary parts of the reconstructed density matrices for ( a ) and ( d ) no obstruction, ( b ) and ( e ) obstruction placed 5 mm from the crystal, and ( c ) and ( f ) obstruction placed 45 mm from the crystal. It is clear that the density matrix recovers to the original unobstructed form for a two-dimensional state as well as higher-dimensional states. The density matrices were calculated by measuring an over-complete set of modes and applying a maximum-likelihood estimation using a least-squares fit to the measurements. This optimization technique ensures a density matrix with non-negative eigenvalues and a trace of unity. Full size image From the density matrices, the concurrence of the state was calculated. Concurrence is a measure of entanglement, with a range from 0 (no entanglement) to 1 (maximally entangled) [38] . The concurrence can only be calculated for two-dimensional subspaces, so we considered two different OAM subspaces, | ℓ =±2› and | ℓ =±4›, to demonstrate that the self-healing property holds for higher OAM modes. The unobstructed BG mode for subspace | ℓ =±2› (| ℓ =±4›) generated an average quantum contrast (see Methods) of QC =43.2±2.0 ( QC =41.7±2.0) and a concurrence of C =0.95±0.02 ( C =0.94±0.02). When the obstruction was placed 5 mm from the crystal, the concurrence dropped to C =0.40±0.02 ( C =0.43±0.02), but recovered to a value of C =0.94±0.02 ( C =0.91±0.02) at 50 mm from the crystal. The results for the coincidences, quantum contrast and concurrence of the | ℓ =±2›-entangled photons are shown in Fig. 8a–c , respectively. All three graphs display similar trends, where the values increase after a minimum distance represented by the yellow dashed line. As in the classical case, where energy is lost in the recovered field, the coincidence counts also do not fully recover to the original unobstructed rate. Consequently, the recovered quantum contrast does not return to the unobstructed value, as the accidental count rate remains fairly constant with the insertion of the obstruction. 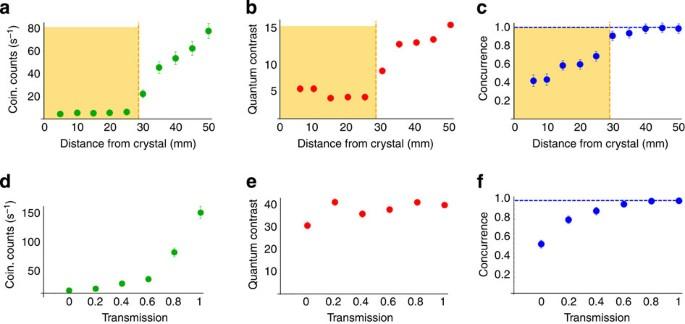Figure 8: Comparison between an obstructed and attenuated beam. Measurements of the coincidence count rate, quantum contrast and concurrence of obstructed (a–c) and attenuated (d–f) entangled photons for |ℓ=±2›. The obstruction was moved in 5 mm intervals along the propagation axis, at which the measurements were recorded. The dashed yellow line representszmin, the calculated distance at which recovery is expected (recovery is not expected within the yellow shaded region). A polarizer was rotated to attenuate the coincidence count rate and vary the degree of transmission from 0 (background levels) to 1 (unattenuated and unobstructed). The coincidence count rates and quantum contrast represent the average of 10 measurements. The average error for the concurrence is ±0.01, which is calculated by generating additional data sets by addingfluctuations to the measured coincidence countsCiand then repeating the concurrence calculations described in the text. The unobstructed concurrence value is represented by the blue dashed lines. Figure 8: Comparison between an obstructed and attenuated beam. Measurements of the coincidence count rate, quantum contrast and concurrence of obstructed ( a – c ) and attenuated ( d – f ) entangled photons for | ℓ =±2›. The obstruction was moved in 5 mm intervals along the propagation axis, at which the measurements were recorded. The dashed yellow line represents z min , the calculated distance at which recovery is expected (recovery is not expected within the yellow shaded region). A polarizer was rotated to attenuate the coincidence count rate and vary the degree of transmission from 0 (background levels) to 1 (unattenuated and unobstructed). The coincidence count rates and quantum contrast represent the average of 10 measurements. The average error for the concurrence is ±0.01, which is calculated by generating additional data sets by adding fluctuations to the measured coincidence counts C i and then repeating the concurrence calculations described in the text. The unobstructed concurrence value is represented by the blue dashed lines. Full size image From the high-dimensional density matrices in Fig. 7 , we calculated the fidelity of the states. Fidelity is a measure of how close the measured state is to a maximally entangled state, where a perfectly entangled state will have a fidelity of unity with the maximally entangled state. We have extended this demonstration to higher dimensions by reconstructing the density matrices for dimension d =4, where | ℓ ={−2, −1, 1, 2}›. The reconstruction process via full-state tomography is time consuming and thus only one high-dimensional state was chosen. The density matrices for different placements of the obstruction are shown in Fig. 7d–f . Table 1 shows the fidelity measurements recorded at different positions of the obstruction from the crystal. Table 1 Measured fidelity at different obstacle positions from the crystal. Full size table The measured fidelities for both dimensions recover to their relative unobstructed values. Fidelity decreases as the state dimension increases, however, the recovered fidelity for d =4 lies above the threshold states, which are defined by the minimum probability for which a high-dimensional Bell inequality is violated [39] . We have therefore demonstrated that the self-healing property of Bessel beams, even when applied to single photons, can overcome the losses associated with an obstruction, allowing sufficient measurement of the spatial correlations to reveal the quantum entanglement of the photon pairs. Our results show that by making projective measurements in the BG basis, we were able to recover the reduction in the measured degree of entanglement resulting from the losses introduced by the obstruction. By comparison, when the LG measurement basis is chosen, the entanglement is not recovered. From the density matrices, we see that while the obstruction perturbs the system, when measured beyond the minimum self-healing distance, the density matrix reverts to the original unobstructed form. Comparing the graphs of the coincidence count rates and concurrence in both experiments, we observe a similar trend: the degree of entanglement is low for low coincidence count rates and then increases with the count rate. It appears that the off-axis obstruction does not destroy the entanglement by scattering a particular OAM state into many OAM states, as observed in turbulence-related experiments [20] , but rather decreases the measured degree of entanglement by reducing the two-photon count rates to background levels. For completeness, we also measured the response of an unobstructed BG mode in the presence of attenuation. By rotating a polarizer in the path of the down-converted light the transmission of the photons could be varied from background levels (≈0 transmission) to normal conditions (transmission of 1). The coincidence count rate, quantum contrast and concurrence for various transmission values are shown in Fig. 8d–f , respectively. The quantum contrast ( Fig. 8b ) suggests that the obstacle blocks one of the entangled photons, thus diminishing the coincidence rate but maintaining a high single-photon count rate. However, the attenuated quantum contrast remains fairly constant unlike that of the obstructed beam. The attenuation reduced the count rates for both the single and coincidence counts proportionally, thereby maintaining a constant quantum-contrast ratio. The obstruction on the other hand reduced only the coincidence count rate and in turn the quantum contrast. The entanglement is therefore obscured by the noise. The correlations are recovered beyond the minimum distance after the obstacle because the mode itself recovers, thus increasing the signal at the detector because of an improved overlap between the hologram and the projected mode. Interestingly, the measurement choice is made after the photons have encountered the obstacle. By contrast, in a classical experiment, the mode is chosen or generated before interacting with the obstacle. In conclusion, we have exploited the self-healing property of BG modes in a quantum entanglement experiment to recover the reduction in the measured degree of entanglement. We showed that the coincidence count rate is reduced in the presence of an obstacle, but that the count rate recovers after a particular distance owing to the self-healing feature of BG modes. This trend was similarly reported for the degree of entanglement of the quantum state, where the concurrence of the obstructed mode returned to its original, unobstructed value. These results may be useful for quantum key distribution and quantum communication systems, where preservation of entanglement over long distances and in the presence of an obstruction is crucial. Experimental details The laser source was a mode-locked ultraviolet laser (Vanguard 355–2500) with a modal diameter of 1 mm, producing pulses of ~10 ps at a repetition rate of 80 MHz. The BBO crystal was cut at 33° to produce collinear, frequency-degenerate down-converted photon pairs at 710 nm. The crystal was tilted to produce near-collinear down-conversion. An interference filter or bandpass filter centred at 710 nm was used to reflect the pump light and transmit the down-converted photon pairs. The variable aperture acted as a spatial filter of the higher-order diffraction modes. The projective measurements were performed by the HoloEye Pluto SLMs (1,080 × 1,920 pixels), which have a resolution of 8 μm per pixel and were calibrated for near-infrared wavelengths. Additional interference filters were placed before the SMFs to select only the photons at 710 nm. Each SMF has a modal radius of 2.3 μm. The Perkin Elmer APDs have a dark count of 200 s −1 , which were connected to a coincidence counter with a gating time of 12.5 ns. The back-projection experiment made use of a 705-nm diode (Laser 2000), temperature tuned to 710 nm. The images of the obstructed beams were captured on a CCD camera. CHSH S parameter The CHSH-Bell parameter, as defined in Leach et al. [35] , is given by where with C ( θ A , θ B ) being the coincidence count rate for the particular orientation of each hologram. By calculating the propagation of uncertainty, we were able to compute a s.d. for the S parameters. Calculating quantum contrast Quantum contrast is a ratio of the coincidence count rate with the accidental count rate. The accidental count rate is defined as S A S B Δ t , where S A,B is the single-count rate in arm A(B) and Δ t is the gating time of the coincidence counter. Thus we can write the quantum contrast as QC = C / S A S B Δ t , where C is the coincidence count rate. Calculating concurrence The concurrence is given by C ( ρ )=max{0, λ 1 − λ 2 − λ 3 − λ 4 }, where λ i are the eigenvalues, in decreasing order, of the Hermitian matrix , where is the spin-flipped state of the density matrix ρ . The qubit OAM density matrices consist of 16 elements, which were calculated by performing a full-state tomography, consisting of 36 projective measurements. That is, the probability of simultaneously finding each of the photons (in the entangled pair) in one of six non-orthogonal states was measured. Although only 16 measurements are required to reconstruct the two-dimensional density matrix, the over-complete 36 measurements allow a least-squares fit to be performed. Calculating fidelity The fidelity is defined as which is a measure of how close our d -dimensional reconstructed state, ρ d , is to the target state ρ T =| ψ T ›‹ ψ T |. In our case the target state is the (pure) maximally entangled state, | ψ T ›= | ℓ › s |− ℓ › i , where ℓ ranges over d different values and c ℓ =1/ represents the expansion coefficients. How to cite this article: McLaren, M. et al. Self-healing of quantum entanglement after an obstruction. Nat. Commun. 5:3248 doi: 10.1038/ncomms4248 (2014).